Enhancing droplet deposition throughin-situprecipitation Retention of agricultural sprays on plant surfaces is an important
challenge. Bouncing of sprayed pesticide droplets from leaves is a major source of
soil and groundwater pollution and pesticide overuse. Here we report a method to
increase droplet deposition through in-situ formation of hydrophilic surface defects that can arrest droplets during impact. Defects are created by simultaneously spraying oppositely charged polyelectrolytes
that induce surface precipitation when two droplets come into contact. Using
high-speed imaging, we study the coupled dynamics of drop impact and surface
precipitate formation. We develop a physical model to estimate the energy
dissipation by the defects and predict the transition from bouncing to sticking. We
demonstrate macroscopic enhancements in spray retention and surface coverage for
natural and synthetic non-wetting surfaces and provide insights into designing
effective agricultural sprays. Sprays are used in a wide range of applications, including
agriculture, paints, coatings, cosmetics and medicine. In agriculture, sprays are
the most common means to deliver pesticides, some nutrients and other chemicals to
plants [1] , [2] , [3] . Some of these chemicals, especially pesticides,
are toxic, and there is an increasing demand to reduce their
use [4] . A
study found that pesticides could be detected 90% of the time in agricultural
streams, 50% in shallow wells and 33% in major deep aquifers across the
USA [5] . Therefore, there is a significant need to eliminate or substantially reduce the
sources of deposition inefficiencies in sprays. One of the most important
inefficiencies arises from the low retention of sprayed liquids on plant surfaces
due to their hydrophobic/superhydrophobic properties—droplets from sprays impacting
plant surfaces can bounce or roll off plant surfaces. Such plants are common, and
they usually get their non-wetting properties from the presence of waxy features on
their surface [6] , [7] , [8] . As a result, most of the liquid from agricultural
sprays ends up in the soil, polluting it and contaminating
groundwater [9] , [10] . Similarly, low retention of sprayed water leads to significant water consumption in
frost protection of plants [3] . The impact of a liquid droplet on a solid surface has been extensively
studied [11] , [12] , [13] , [14] , [15] , [16] , [17] , [18] , [19] , [20] , [21] , [22] , [23] . It is known that for a hydrophobic surface, at moderate impact velocities, the
droplet undergoes an expansion phase, driven by inertial forces, followed by a
retraction phase, driven by surface tension, that may lead to a bounce-off. The
outcome of the impact, whether the droplet adheres or bounces off, depends on
multiple factors related to the surface and sprayed liquid. The relevant surface
properties are surface energy and surface texture and the drop parameters are
surface tension, viscosity and size. Current approaches to improve droplet
deposition rely on modifying the fluid properties in a way that enhances
retention [6] , [24] , [25] . One common approach to improve drop retention is to add surfactants to
the sprayed liquid in order to reduce the surface tension and promote spreading of
droplets on the surface [26] . However, even if surfactants enhance spreading in
the static case, their effect in a dynamic impact process is more complex. Surfactant molecules must diffuse from the bulk to the newly formed interfaces, as
the drop undergoes dramatic changes in shape. If the timescale of this diffusion is
higher than the contact time of the droplet with the solid—that is, the time a
droplet spends on the surface before bouncing [18] , [27] , these surfactants will have a smaller effect. Therefore, the appropriate parameter to study is the dynamic surface tension, and,
considering these dynamic effects, the role of surfactants in drop retention has
been shown to be less pronounced than anticipated [28] , [29] . Moreover, adding surfactants leads to smaller
droplets in sprays, which aggravate other problems such as wind drift and
evaporation [30] . Another recent approach is based on modifying the rheological
properties of the fluid by adding small amounts of a polymer additive to the sprayed
solution [25] , [31] . It has been shown that these dilute polymer solutions delay the retraction phase and
lead to the deposition of the droplet. For small amounts of polymer, the viscosity
and surface tension of the solution remain approximately the same as water. It was
suggested that the observed retention arises from non-Newtonian properties,
particularly the extensional viscosity of the polymer solution η e . Stretching the fluid during
expansion and retraction unfolds and deforms high molecular weight polymers leading
to significant energy dissipation that can prevent droplet rebound. Improvements in
deposition on different surfaces have been reported. However, the underlying
physical mechanism is still being investigated [32] , [33] , [34] . Here we propose an alternate approach to enhance drop retention by
altering the target surface properties in-situ during the spray process by forming sparse hydrophilic defects onto the substrate. These defects would act to pin the contact line of impinging droplets and suppress
bouncing [35] . Inspired by the layer-by-layer deposition
techniques [36] , [37] (though this is a different concept), we create these pinning defects by adding
small quantities of oppositely charged polyelectrolytes to separate solutions and
spraying them simultaneously using two nozzles, as shown schematically in Fig. 1a . When droplets containing
oppositely charged polyelectrolytes come into contact, a precipitation reaction
occurs and results in the formation of hydrophilic surface defects that pin the drop
to the surface and enhance retention ( Fig. 1b ). After demonstrating the concept with spray experiments, we
study the possible interactions between droplets of the oppositely charged
polyelectrolyte solutions by performing individual drop-on-drop experiments and
observing the deposited precipitate on the surface through microscopy. We then
derive a criterion predicting the transition between bouncing and sticking for two
impacting droplets and define a characteristic non-dimensional number for this
problem. We finally translate these individual droplet results to sprays and show
that simultaneous spraying of polyelectrolyte solutions on synthetic and natural
superhydrophobic surfaces leads to a substantial increase in the deposition and
retention of the liquid. 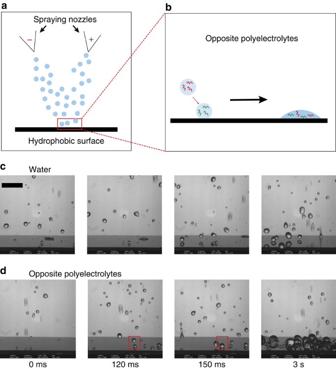Figure 1: Simultaneous spraying of opposite polyelectrolytes. (a) Schematic of experimental
set-up for simultaneous spraying of opposite polyelectrolytes. (b) Expected behaviour for the impact of a droplet
with one polyelectrolyte polarity on a droplet with an oppositely charged
polyelectrolyte. The coalesced drop sticks to the surface. (c,d) Snapshots of
simultaneous spraying on a superhydrophobic surface. Sprays with very low
droplet density were used to enhance visualization and slow down the
process. In the first row, the two sprayers are spraying water and the
surface remains dry. Almost all droplets bounce off. Some small droplets are
deposited but they are cleared as soon as another droplet impacts them (seeSupplementary Movie 1). In
the second row, opposite polyelectrolytes are sprayed. Individual droplets
hitting the surface still bounce off. After 120 ms of spraying, the first
event of a droplet of one polyelectrolyte hitting a droplet containing the
opposite polyelectrolyte occurs. The coalesced drop sticks to the surface.
Subsequent drops that hit this droplet also coalesce on it. Similar events
happen all over the surface. Many droplets can be seen on the surface after
3 s of spraying (seeSupplementary Movie
2). Scale bar, 1 cm. Figure 1: Simultaneous spraying of opposite polyelectrolytes. ( a ) Schematic of experimental
set-up for simultaneous spraying of opposite polyelectrolytes. ( b ) Expected behaviour for the impact of a droplet
with one polyelectrolyte polarity on a droplet with an oppositely charged
polyelectrolyte. The coalesced drop sticks to the surface. ( c , d ) Snapshots of
simultaneous spraying on a superhydrophobic surface. Sprays with very low
droplet density were used to enhance visualization and slow down the
process. In the first row, the two sprayers are spraying water and the
surface remains dry. Almost all droplets bounce off. Some small droplets are
deposited but they are cleared as soon as another droplet impacts them (see Supplementary Movie 1 ). In
the second row, opposite polyelectrolytes are sprayed. Individual droplets
hitting the surface still bounce off. After 120 ms of spraying, the first
event of a droplet of one polyelectrolyte hitting a droplet containing the
opposite polyelectrolyte occurs. The coalesced drop sticks to the surface. Subsequent drops that hit this droplet also coalesce on it. Similar events
happen all over the surface. Many droplets can be seen on the surface after
3 s of spraying (see Supplementary Movie
2 ). Scale bar, 1 cm. Full size image Spray experiments To study the effect of precipitation on drop impacts, we used two
polyelectrolyte molecules. Linear polyethyleneimine was the positively charged
polyelectrolyte, with NH 2 + groups in solution, while polyacrylic acid was the negatively charged
polyelectrolyte with COO − groups in solution. The molecular weight of both polyelectrolytes was ∼ 20,000 g mol −1 . These polyelectrolytes were
dissolved in water at different concentrations. Separately, the polyelectrolyte
solutions are very dilute and have physicochemical properties that are close to
pure water. In particular, surface tension of all the used solutions was measured
to be within 13% of that of water ( Supplementary
Fig. 1 ). The electrical interactions between ions in solution depend on their zeta potential, which is a measure of the electrical potential difference between the layer of fluid attached to a molecule or particle and the bulk of the solution. The zeta potential of polyelectrolytes depends on the pH of the solution, and, for our experiments, we chose a pH ∼ 4.5 for which both potentials are sufficiently high to have a substantial interaction between the two polyelectrolytes [38] , [39] . At this pH ∼ 4.5, we observed that mixing solutions of these two polyelectrolytes resulted in spontaneous formation of insoluble precipitates in the solution [40] , [41] . The precipitates were observed as whitish
residues, and they were formed both in the bulk of the solution and on the surface
on which the liquid was deposited. We observed that the surface precipitates are
hydrophilic and can strongly pin impinging droplets during impact. A silicon nanograss surface composed of random features of typical
size and spacing around 200 nm and coated with a hydrophobic modifier was used as
a model superhydrophobic surface in this study. For this surface, we measured a
contact angle of 165° and a contact angle hysteresis smaller than 5° (ref. 42 ). Simultaneous spraying of water
droplets with and without polyelectrolytes was performed on these surfaces and the
interaction was captured using a high-speed camera ( Fig. 1c,d Supplementary Movies 1 and 2 ). Sparse
sprays were used for better visualization as they slowed down the rate of defect
formation. When pure water droplets are sprayed, they bounce off the surface as
expected and the surface remains clear as shown in Fig. 1c . Some small droplets may stick to the surface, but as soon as
they are impacted by another impinging droplet, they bounce off. In contrast,
spraying water droplets containing oppositely charged polyelectrolytes increases
liquid retention as shown in Fig. 1d . Close inspection of the spray ( Supplementary Movie
2 ) reveals that not all droplets impacting the surface lead to
retention. When single droplets impact the surface they bounce off similar to pure
water droplets. Further experiments with impacts of single droplets of either
polyelectrolyte show that they bounce off ( Supplementary Fig. 2 ), and spraying only one of the polyelectrolyte solutions results in no retention. Therefore, the retention in simultaneous spraying must come from the interaction between at least two droplets. Indeed, when multiple droplets collide on the surface, the coalesced drop is arrested. The drop is then anchored at the surface and does not detach even when additional droplets impinge on it. The anchored drop continues to grow due to the coalescence of subsequent impacting droplets. As time progresses, the surface is covered with many anchored drops that continue to grow and, after ∼ 3 seconds of spraying, much of the surface is covered with liquid. We notice that the most frequent case for two-droplet interactions is when small single droplets stay on the surface upon impact and are subsequently impacted by another impinging drop. Thus, we choose drop-on-drop impact experiments as our model experiments. Drop-on-drop impacts In Fig. 2 , we present the
five possible cases of two-droplet interactions: A positive droplet (linear
polyethyleneimine) impinging on another positive one, a negative droplet
(polyacrylic acid) impinging on a negative one, a positive and negative droplet
colliding and coalescing in midair and then impinging on the surface, a positive
droplet impinging on a negative one and a negative droplet impinging on a positive
one. For each of these cases, the drop-on-drop impact experiment is filmed with a
high-speed camera at 10,000 frames per second and the impact location of the dried
surface is imaged using a scanning electron microscope (SEM). 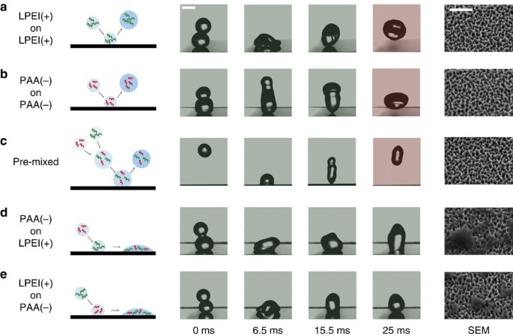Figure 2: Possible droplet interactions in simultaneous spraying of opposite
polyelectrolytes. The first column contains schematics of the five possible
scenarios. The next columns are snapshots of individual drop impacts for
each of the previous scenarios. The rightmost column contains SEM images
of the surface after the impacts. The images were taken at a tilt angle of
30°. Only the last two cases result in arresting the droplet and leaving a
residue on the surface. (a) A 2 mm
droplet of linear polyethyleneimine (LPEI) is deposited on the
superhydrophobic surface and another LPEI droplet impacts it vertically.
Snapshots of the impact show a similar behaviour to typical single droplet
impacts: Upon coalescence the merged droplet expands then retracts and
eventually bounces off the surface. The process lasts around 20ms, which
is comparable to the contact time of single impinging droplets of similar
radius. The SEM image shows the features of the surface, uncovered, as
they were before the impact. (b) The
polyacrylic acid (PAA) on PAA impact exhibits a similar behaviour and
results in an unspoiled surface as well. (c) LPEI and PAA solutions are premixed, forming a bulk
precipitate. The impact of a droplet of this mixture on a superhydrophobic
surface results in bouncing, with no satellite droplet left behind. SEM
images show that nothing is deposited on the surface. The precipitates
seem to remain in the bulk and not act as a pinning site on the surface.
(d) When a PAA drop impacts an LPEI
drop, after a similar expansion phase, the retraction phase ends with an
arrested droplet. The SEM image shows the deposition of a residue on the
surface, formed by the precipitation of the opposite polyelectrolytes when
the two droplets merged on the surface. For complete movie, seeSupplementary Movie 3.
(e) LPEI on PAA is similar and leads to
the droplet sticking on the surface. Scale bar, 2 mm (snapshots). Scale
bar, 2μm (SEM). Figure 2: Possible droplet interactions in simultaneous spraying of opposite
polyelectrolytes. The first column contains schematics of the five possible
scenarios. The next columns are snapshots of individual drop impacts for
each of the previous scenarios. The rightmost column contains SEM images
of the surface after the impacts. The images were taken at a tilt angle of
30°. Only the last two cases result in arresting the droplet and leaving a
residue on the surface. ( a ) A 2 mm
droplet of linear polyethyleneimine (LPEI) is deposited on the
superhydrophobic surface and another LPEI droplet impacts it vertically. Snapshots of the impact show a similar behaviour to typical single droplet
impacts: Upon coalescence the merged droplet expands then retracts and
eventually bounces off the surface. The process lasts around 20ms, which
is comparable to the contact time of single impinging droplets of similar
radius. The SEM image shows the features of the surface, uncovered, as
they were before the impact. ( b ) The
polyacrylic acid (PAA) on PAA impact exhibits a similar behaviour and
results in an unspoiled surface as well. ( c ) LPEI and PAA solutions are premixed, forming a bulk
precipitate. The impact of a droplet of this mixture on a superhydrophobic
surface results in bouncing, with no satellite droplet left behind. SEM
images show that nothing is deposited on the surface. The precipitates
seem to remain in the bulk and not act as a pinning site on the surface. ( d ) When a PAA drop impacts an LPEI
drop, after a similar expansion phase, the retraction phase ends with an
arrested droplet. The SEM image shows the deposition of a residue on the
surface, formed by the precipitation of the opposite polyelectrolytes when
the two droplets merged on the surface. For complete movie, see Supplementary Movie 3 . ( e ) LPEI on PAA is similar and leads to
the droplet sticking on the surface. Scale bar, 2 mm (snapshots). Scale
bar, 2μm (SEM). Full size image The results in Fig. 2 show
that the impacts involving two droplets containing the same polyelectrolyte result
in bouncing in a sequence of spreading and retraction phases that is similar to
the impact of a single droplet ( Fig. 2a,b ). The measured contact time is also close to that of a single
droplet (within 15%), and no deposits can be seen in the SEM images. Forming the
precipitates beforehand by premixing positive and negative polyelectrolytes before
impact does not cause droplets to stick to the surface. None of the bulk
precipitates remain on the surface as shown in Fig. 2c . Thus, spraying a solution containing pre-formed precipitates
does not increase the liquid retention. The same bouncing behaviour is observed
when other hydrophilic particles are added to the droplet. As shown in Supplementary Fig. 3 , droplets
containing 3 μm silica particles bounce off superhydrophobic surfaces without
leaving any particle residue. However, drop-on-drop impacts of droplets with
oppositely charged polyelectrolytes lead to droplets sticking to the surface. The
droplets are arrested by the pinning sites that are formed due to the in-situ precipitation of oppositely charged
polyelectrolytes on the surface ( Fig. 2d,e ). Studying these different cases confirms that the in-situ formation of surface precipitates is the key to
enhanced retention and explains what happens when oppositely-charged
polyelectrolyte solutions are sprayed: Sufficiently small droplets of one solution
may stick to the surface when pinning forces due to the natural hysteresis of the
surface overcome inertial forces. Upon impact with another incoming droplet, the
coalesced drop will only stick if the two droplets contain oppositely charged
polyelectrolytes and can react to form additional surface pinning sites that
arrest the coalesced drop. When two droplets containing oppositely charged polyelectrolytes
coalesce, there are oppositely charged macromolecules in solution. When these
molecules are in close proximity such that the electrical charges are not completely
screened, they are attracted to each other and subsequently attract other molecules
to form precipitates, as shown in Fig. 3a . Molecules that are close to the surface may be attracted to the
surface [43] and serve as a nucleation site for a surface
precipitate. These precipitates act as defects and pin the contact line of the
retracting droplet. This pinning dissipates energy and can prevent the droplet from
bouncing. As shown in the top view images in Fig. 3b , the retraction front in the case of water droplets is
predominantly axisymmetric due to minimal pinning. However, for positive on negative
polyelectrolyte drop impact the retracting front is composed of multiple sharp
corners and filaments, indicating contact line pinning (see Supplementary Movie 4 ). 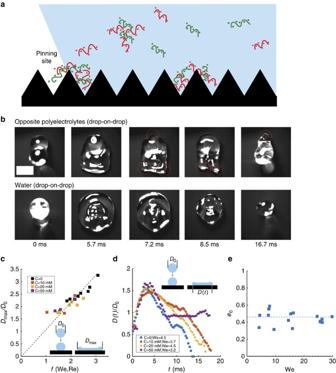Figure 3: Defects formation and drop-on-drop impact dynamics. (a) Schematic of the formation of
precipitates in the liquid and the role of surface precipitates in pinning
the receding contact line of a droplet. (b)
Top view snapshots of drop-on-drop impacts. Water droplets exhibit an
axisymmetric uniform retraction, while, for polyelectrolytes, retraction is
asymmetric and comprises sharp edges, which are the signature of pinning
locations (red circles). For complete movie, seeSupplementary Movie 4. Scale bar, 2 mm.
(c) Normalized maximum diameter as a
function of the correlation functionf(We, Re). The Weber number spanned an order of magnitude (4–40)
and was varied by using two droplet sizes (1.1 and 1.9 mm radius) and four
impact velocities for each. (d) Normalized
contact length as a function of time for four scenarios. All droplets
expand, reach a maximum diameter then retract. Bouncing occurs in three
cases where the spreading coefficient goes to zero, while sticking occurs in
the case with the highest polyelectrolyte concentration C. (e) Restitution coefficient as a function of the
impact Weber number for water. The Weber number was varied by changing the
droplet size and the impact velocity. In all drop-on-drop experiments, both
drops had the same size. Figure 3: Defects formation and drop-on-drop impact dynamics. ( a ) Schematic of the formation of
precipitates in the liquid and the role of surface precipitates in pinning
the receding contact line of a droplet. ( b )
Top view snapshots of drop-on-drop impacts. Water droplets exhibit an
axisymmetric uniform retraction, while, for polyelectrolytes, retraction is
asymmetric and comprises sharp edges, which are the signature of pinning
locations (red circles). For complete movie, see Supplementary Movie 4 . Scale bar, 2 mm. ( c ) Normalized maximum diameter as a
function of the correlation function f (We, Re). The Weber number spanned an order of magnitude (4–40)
and was varied by using two droplet sizes (1.1 and 1.9 mm radius) and four
impact velocities for each. ( d ) Normalized
contact length as a function of time for four scenarios. All droplets
expand, reach a maximum diameter then retract. Bouncing occurs in three
cases where the spreading coefficient goes to zero, while sticking occurs in
the case with the highest polyelectrolyte concentration C. ( e ) Restitution coefficient as a function of the
impact Weber number for water. The Weber number was varied by changing the
droplet size and the impact velocity. In all drop-on-drop experiments, both
drops had the same size. Full size image To further characterize these drop-on-drop impacts, we first measure
the normalized maximum diameter, defined as the diameter of the coalesced droplet
when it reaches its maximal expansion divided by the initial diameter of one droplet D 0 . Figure 3c shows the normalized maximum diameter for
various drop sizes, impact velocities, and polyelectrolyte concentrations. We find
that for our experimental conditions (4<We<40, 500<Re<5000), the
normalized maximum diameter scales as , where We is the Weber number and Re is the Reynolds number, as
was shown in previous studies for single drop impacts [44] , [45] . The results are identical for the cases with
and without polyelectrolytes. Figure 3d shows the time evolution of the normalized contact length D(t)/D 0 for different polyelectrolyte
concentrations. We observe that, similar to the normalized maximum diameter, the
expansion time, defined as the time till the coalesced droplet reaches its maximum
expansion, is not affected by the addition of polyelectrolytes since the contact
line does not encounter any surface defects in the expansion phase. The droplet behaves differently in the retraction phase. Figure 3d shows that increasing the polyelectrolyte
concentration increases the contact time, which becomes infinity for high
concentrations, as the droplet sticks to the surface. It has been shown earlier that
the retraction rate for single drop impacts is a material property and does not depend
on the impact velocity [29] , [46] . We plot the retraction rate in Supplementary Fig. 4 for drop-on-drop impacts with various drop sizes, impact
velocities and polyelectrolyte concentrations. We observe that the retraction rate
does not depend on the impact velocity, similar to the case of single drop
impacts [29] , [46] , and decreases with
polyelectrolyte concentration. The decrease in retraction rate arises from the pinning of the
contact line on the defects formed by polyelectrolyte precipitation. The contact
line may get pinned and depinned several times during the retraction phase, and each
of these events dissipates some energy and slows the retraction. The final outcome
of the impact depends on how much energy is dissipated by pinning and depinning. We
observe that for low concentrations of polyelectrolytes, bouncing might still occur,
while for higher concentrations droplets are arrested. Defect density, and thus the
ability to arrest impacting droplets, intuitively increases with concentration. The
objective is then to find the minimum concentration for which the number of
generated defects arrests the impacting droplets on the surface. To determine this
minimum concentration, we consider the energy balance during impact. Viscous effects
are weak here as the Ohnesorge number [47] . An impacting droplet striking a non-wetting surface will rebound
if enough of its initial kinetic energy, which is converted into surface energy
during the expansion phase, is recovered during the retracting
phase [27] . Since viscous dissipation is negligible, the only mechanism for the droplet to lose
energy is through the pinning forces on the surface. However, part of the initial
kinetic energy is also converted into internal vibration energy due to droplet
oscillations [48] , [49] , [50] . We estimate the fraction of
the initial kinetic energy that gets converted into vibration energy as (1− e 0 2 ) E k where e 0 is the restitution coefficient for the base
case of drop-on-drop impacts of pure water droplets, where there is negligible
pinning [51] . The restitution coefficient is calculated as , where m i , m b are the masses of the droplet and v i , v b are the velocities of the center of mass
before and after impact (here m b / m i =2). As shown in Fig. 3e , despite some scatter in the data, we find that the
restitution coefficient of pure water droplets does not strongly depend on the Weber
number of the impacting droplet and is on the order of 0.4 for our impact
experiments. Assuming that the internal vibration of the droplets is not
significantly affected by polyelectrolytes, this measured restitution coefficient
for water droplets can be used to estimate the vibration energy of polyelectrolyte
droplets. Hence, polyelectrolyte droplets will stick to the surface if the work of
pinning during the retraction phase exceeds the remaining kinetic energy e 0 2 E k . In quantitative terms, the initial kinetic energy of the droplet is E k ∼ ρR 3 V 2 , and the work of pinning on one single
defect is W ∼ σl 2 , where R is the radius of the droplet, V is its impact velocity, ρ is the density, σ is the surface tension and l is the defect size [52] , [53] , [54] . The total work of pinning during the receding phase is then W ∼ σl 2 N defects , where N defects is the total number of
defects under the droplet during the impact. We can then define an average surface
concentration of defects C s , and W ∼ σl 2 R 2 C s . The ratio of kinetic energy
and the work of pinning gives the characteristic non-dimensional number for this
problem, the pinning number , which should govern the transition between bouncing and
sticking. The surface concentration of defects is hard to estimate, and can
vary from zero to a maximal value corresponding to the case where all the
polyelectrolytes in both droplets react and form surface precipitates. In an attempt
to have an expression of Pi as a function of the controlled parameters of the
problem, we make the following hypothesis: the number of surface defects is a
fraction of the total number of defects that can be created by all the
polyelectrolytes in the droplet , where C is defined as the
volumetric molar concentration of monomers and ϕ is the fraction of polyelectrolytes that precipitated during the impact, which can
be estimated, for short contact times, as the ratio of the contact time to the
precipitation time. The pinning number is then To estimate Pi, we use SEM images to estimate the average defect size l , which was around 500 nm. To estimate the
number of monomers per defect, we relate the radius of a semi-flexible polymer chain
to the number of its monomers, using the standard Flory theory, which gives l ∼ aN υ ,
where l is the defect size and a is the monomer size ( ∼ 1 nm) (ref. 55 ). In the case of polyelectrolytes, υ =(3)/(5), and this leads to a number N on the order 10,000 monomers per defect. To determine the ratio ϕ , we
compare the precipitation time to the contact time. As diffusion effects are
negligible during contact time ( τ diffusion ≫ τ contact ), in our experiments, precipitation is
mainly driven by mixing of the droplets. When the two droplets coalesce, they need
some time to completely mix, as shown schematically in Supplementary Fig. 5a . During the mixing phase,
only a fraction of the polyelectrolyte molecules have come into contact with each
other and are able to interact. The mixing is driven by inertial and capillary
forces and the mixing time scales as (refs 56 , 57 ). The precipitation rate then
scales as . We experimentally measured the precipitation rate of two
coalescing droplets with opposite polyelectrolytes, which was indeed found to scale
as as predicted (See Supplementary
Note 1 and Supplementary Fig. 5 for details). The contact time has the same scaling law as the
mixing time , but with a different pre-factor [27] . Thus, we expect ϕ to be independent of the drop parameters and only
depend on the ratio of the pre-factors. The experimentally measured pre-factor is
larger for the mixing time than for the contact time by about an order of magnitude,
so . We performed several drop-on-drop impact experiments, varying the
concentration, radius and velocity, and recorded whether the outcome was bouncing or
sticking. In Fig. 4 , we can see that for
high kinetic energies, or high Pi, droplets bounce, while they tend to stick for
lower Pi. The transition occurs at a pinning number of around 0.1. Our model of Pi
remains a first-order attempt to capture the physics of the phenomenon, and more
detailed studies on the coupling between precipitation and impact dynamics and their
effect on the size and density of defects are needed to refine the model. 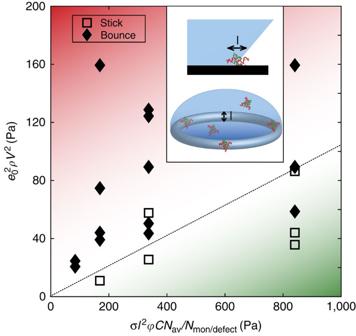Figure 4: Bouncing-Sticking transition in a two-drop impact. The data points are experimental outcomes of impacts at different concentrations, radii and impact velocities. The figure axes are the work of pinning and the kinetic energy of the droplet. The dashed line roughly indicates the transition between bouncing and sticking and corresponds to Pi∼0.1. Below the dashed line, pinning forces are larger than inertia and pinning of the droplet is expected, while bouncing is expected above. The inset illustrates the defect size, and the region around the contact line that is acted upon by pinning forces at a certain time. Figure 4: Bouncing-Sticking transition in a two-drop impact. The data points are experimental outcomes of impacts at different concentrations, radii and impact velocities. The figure axes are the work of pinning and the kinetic energy of the droplet. The dashed line roughly indicates the transition between bouncing and sticking and corresponds to Pi ∼ 0.1. Below the dashed line, pinning forces are larger than inertia and pinning of the droplet is expected, while bouncing is expected above. The inset illustrates the defect size, and the region around the contact line that is acted upon by pinning forces at a certain time. Full size image Finally, the retention of sprayed liquids was measured for different
surfaces and liquids. Sprayers were used to deliver fixed amounts of liquid to the
surface in the form of jets of fine droplets, at constant jet velocity and cone
angle. Two metrics were used to quantify the retention. First, the mass of the
liquid retained by the sample was measured by weighing the sample after every
spray [58] . Second, we measured the surface coverage, i.e., the area covered by the liquid
divided by the total area of the substrate [59] . The first metric characterizes
how much liquid can stick to the surface, while the second metric quantifies the
uniformity of the coverage. 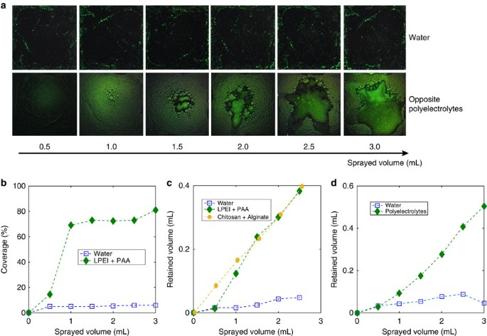Figure 5: Water and opposite polyelectrolytes spraying on a superhydrophobic
surface. (a) Photographs of a 2 × 2”
superhydrophobic surface after spraying fixed volumes of water and
polyelectrolytes (linear polyethyleneimine (LPEI) and polyacrylic acid
(PAA)). A fluorescent dye was added to allow visualization. (b) Coverage of the surface by the liquid in the
same experiments. (c) Retained volume of
liquid on the same surface after spraying water, LPEI+PAA and Chitosan +
Alginate. (d) Retained volume of Chitosan +
Alginate on a lotus leaf. Figure 5a shows images of the
surfaces (2 × 2 inches), as different liquids are sprayed. A fluorescent dye was
added to all the sprayed liquids for better visualization. As expected, for a
superhydrophobic surface, very little water was retained and the coverage did not
exceed 7% after 3 ml were sprayed, as shown in Fig. 5b . However, when oppositely charged polyelectrolytes (concentration
20 mM) were simultaneously sprayed on the superhydrophobic surface, much more of the
liquid remained on the surface: the coverage was 70% after 1 ml and reached 80% when
3 ml of liquid were sprayed. The retained volume exhibits similar trends, as shown
in Fig. 5c . When polyelectrolytes are
sprayed, the retained volume continuously increases, and it only stops when the
sample eventually cannot hold more liquid and further spraying removes the excess
accumulated liquid. There is a 10-fold increase in retention as compared with water
and the retained volume is even close to the retained volume of water on a
superhydrophilic surface that we measured in separate experiments ( Supplementary Fig. 6 ), and which provides an
estimate of the maximal attainable value for retention. Figure 5: Water and opposite polyelectrolytes spraying on a superhydrophobic
surface. ( a ) Photographs of a 2 × 2”
superhydrophobic surface after spraying fixed volumes of water and
polyelectrolytes (linear polyethyleneimine (LPEI) and polyacrylic acid
(PAA)). A fluorescent dye was added to allow visualization. ( b ) Coverage of the surface by the liquid in the
same experiments. ( c ) Retained volume of
liquid on the same surface after spraying water, LPEI+PAA and Chitosan +
Alginate. ( d ) Retained volume of Chitosan +
Alginate on a lotus leaf. Full size image Spray experiments with a polyelectrolyte concentration of 2 mM resulted in zero retention while experiments with 20 mM showed large enhancements in retention. These results are consistent with our Pi model, which predicts the transition from bouncing to sticking drops to occur at a concentration of ∼ 10 mM for our sprays. We also show similar retention properties using different
polyelectrolyte molecules. Retained volume using Chitosan (positively charged) and
Alginate (negatively charged) is also largely increased, as shown in Fig. 5c . These polyelectrolytes are polysaccharides
that are non-toxic, biocompatible and biodegradable, which makes them excellent
candidates for plant treatment [60] , [61] , [62] . We finally sprayed these
polyelectrolytes on superhydrophobic lotus leaves and observed a similar pattern of
increased retention ( Fig. 5d ), showing their
efficiency on natural surfaces as well. The method described here is not limited to
superhydrophobic surfaces and works similarly on hydrophobic surfaces ( Supplementary Fig. 7 ), which makes it applicable
to a large variety of plants and surfaces in practice. We demonstrate here a new mechanism to enhance spray deposition on
hydrophobic surfaces through in-situ precipitation of polyelectrolytes on the surface. We show how defects formed in-situ on the surface during the impact can
pin the impinging droplets, and show the advantages of creating these hydrophilic
wetting defects in-situ . We study the mechanism
of precipitate formation in coalescing droplets, which gives insights on the extent
of the precipitation reaction during droplet impacts, and we propose a simple model
balancing kinetic and pinning energies that leads to a criterion characterizing the
transition between bouncing and sticking droplets or sprays. This method allows
surface modification and deposition of the liquid of interest in one single step and
introduces a new control parameter in the design space for sprays, which is the
polyelectrolyte concentration. We show that this method could work on different
surfaces and with different types of polyelectrolytes, as long as their zeta
potential is high enough to interact, and there are several natural, biodegradable
and readily available polyelectrolytes that can be used. It is known that low
retention of pesticides on hydrophobic plants is a major problem in
agriculture [6] . By adding small amounts of these polyelectrolytes
to sprays, the quantity of pesticides used could be significantly reduced, while
coverage is increased, offering full protection to the plant and limiting the toxic
effects of pesticides. This method can also be used for other agricultural sprays,
paints, and any other process that involves sprays or droplet deposition. Fabrication of superhydrophobic surfaces Plasma etch with O 2 and
SF 6 was performed on silicon substrates to make a silicon
nanograss texture. The latter is a superhydrophilic surface with contact angles
around 0°. To make it superhydrophobic, the surface was coated with a hydrophobic
modifier (octadecyltrichlorosilane). Advancing and receding contact angles of
deionized water on a nanograss silicon surface treated with the hydrophobic
modifier were measured with a goniometer (Model 500, ramé-hart) at 25 °C to be
165°±2° and 160°±3°, respectively. Polyelectrolyte solutions Four polyelectrolyte molecules were used. All the polyelectrolytes
were obtained from Sigma- Aldrich and used as received. The properties of the used
solutions are in Table 1 . Table 1 Solutions properties. Full size table The pH was adjusted using HCl and NaOH for all solutions except the
one with chitosan that was adjusted by adding acetic acid. Spraying method An airbrush was vertically fixed, 21 cm above the horizontal
sample. The pressure of the air supply to the airbrush was maintained constant
throughout the whole set of experiments so as to keep the same jet velocity and
cone angle. The liquid was delivered to the airbrush by inputs of 500 μl using a
syringe. The samples (2′′−2′′) were chosen to be bigger than the spray cone (more
than 98% of the sprayed liquid hits the sample). Coverage determination A small quantity of fluorescent dye (Fluorescein sodium salt) was
added to the sprayed solutions. Imaging under ultraviolet light was realized after
each spray, and image processing using ImageJ was performed to determine the
fraction of the surface covered by the liquid. Data availability The authors declare that the data supporting the findings of this
study are available within the article and its supplementary information . How to cite this article : Damak, M. et al . Enhancing droplet deposition through in-situ precipitation. Nat. Commun. 7:12560 doi: 10.1038/ncomms12560 (2016).